Borealin dimerization mediates optimal CPC checkpoint function by enhancing localization to centromeres and kinetochores The chromosomal passenger complex (CPC) localizes to centromeres where it activates the mitotic checkpoint in response to inappropriate inter-kinetochore tension. This error correction function is essential for proper chromosome segregation. Here we define several critical features of CPC localization and function. First, the Borealin dimerization domain suppresses dynamic exchange at the centromere to allow optimal CPC function. Second, Borealin dimerization is essential to target a subpopulation of CPC proximal to the kinetochore when the mitotic spindle is disrupted. This subpopulation is also needed for full CPC checkpoint function. The existence of a pool of CPC at the kinetochore suggests that error correction is more complicated than predicted from the Aurora B phosphorylation gradient model. Finally, Haspin kinase plays a key role in maintaining the slowly exchanging centromere Borealin pool, while Aurora B and Mps1 play minimal roles in maintaining CPC localization once cells are in mitosis. Cancer cells are commonly aneuploid, a condition defined by the gain or loss of whole chromosomes or chromosomal segments [1] , [2] . Aneuploidy can result from errors in cell division, such as mis-segregation of individual chromosomes during mitosis [3] . Therefore, cell division is monitored by multiple cell cycle checkpoints to prevent aneuploidy [4] , [5] . For example, the spindle assembly checkpoint (SAC) prevents anaphase onset until all chromosomes achieve biorientation on the mitotic spindle [6] . The SAC is activated by unattached kinetochores [7] . Anaphase onset is also delayed in response to insufficient tension generated between sister kinetochores, for example, when both kinetochores attach to the same spindle pole. Insufficient tension triggers the release of bound microtubules, generating unattached kinetochores that activate the SAC [8] , [9] . The tension-sensing system that regulates kinetochore–microtubule interactions depends on the chromosomal passenger complex (CPC) [6] , composed of Borealin, Survivin, INCENP and Aurora B [8] . Prior to anaphase, the CPC localizes to inner centromeres, adjacent to sister kinetochores, to monitor inter-kinetochore tension. The prevailing model that explains the role of Aurora B in regulating the SAC posits that under low tension, Aurora B phosphorylates microtubule-binding kinetochore proteins resulting in reduced affinity for microtubules leading to dissociation of kinetochore–microtubule interactions [10] , [11] , [12] , [13] , [14] . As chromosomes become bioriented and sister kinetochores are under high tension, Aurora B is spatially separated from the kinetochore and can no longer destabilize kinetochore–microtubule interactions. According to this spatial gradient model, inner centromere localization of the CPC is paramount for error correction [15] . In yeast, however, INCENP can regulate chromosome segregation independent of centromere localization [16] . CPC localization during metaphase is thought to rely on the intersection of two histone modifications at the centromere. Haspin kinase phosphorylates histone H3 on threonine 3 (pH3 T3 ) along chromosome arms and at centromeres, which is bound by Survivin [17] , [18] . The kinetochore-localized kinase Bub1 phosphorylates histone H2A on threonine 120 (pH2A T120 ) at pericentromeric chromatin, which recruits Sgo1/2 (refs 18 , 19 ). Sgo1/2 can bind CDK1-phosphorylated Borealin, which also contributes to CPC localization to centromeres [18] , [20] . Furthermore, Aurora B regulates pH3 T3 by directly activating Haspin via phosphorylation. Also, both Aurora B and Mps1 regulate Bub1 recruitment to kinetochores [17] , [21] , [22] , [23] . We have analysed CPC localization and function using a combination of Borealin structure–function studies, an FK506-binding protein (FKBP)-mediated dimerization system and kinase inhibitors to deplete known CPC receptors at the centromere. Our results suggest that monomeric CPC interacts transiently with the centromere via binding to pH3 T3 , while dimerization enhances centromere binding to provide optimal CPC function. Selective reduction of pH3 T3 reveals a kinetochore-proximal pool of CPC that partly co-localizes with pH2A T120 , and depends on dimerization for localization. Additional experiments suggest that both the inner centromere and kinetochore-proximal pool of CPC contribute to activation of the SAC. Domains of Borealin required for stable centromere binding Borealin can be divided into three functional regions, the N-terminal alpha helices that interact with Survivin and INCENP (amino acids 15–76), an unstructured central region that contains CDK1 phosphorylation sites required for interaction with Sgo1/2 (amino acids 106–219) and a C-terminal dimerization domain (amino acids 224–280) [24] , [25] , [26] . Since Survivin binds pH3 T3 and Sgo1/2 binds pH2A T120 , both the N-terminal and central regions of Borealin are implicated in centromere targeting of the CPC [17] , [18] , [25] , [27] . We analysed truncated forms of Borealin lacking either the dimerization domain (Borealin 1–221 ) or both the central region and the dimerization domain (Borealin 1–110 ). Immunofluorescence analysis of FLAG-tagged Borealin truncations was performed in cells blocked in mitosis with taxol. Full-length Borealin localized to centromeres with little to no detectable cytoplasmic staining ( Fig. 1a,b ). Both Borealin 1–221 and Borealin 1–110 displayed punctate foci between Hec1-stained kinetochores; however, truncated forms of Borealin showed elevated cytoplasmic staining compared with full-length Borealin ( Fig. 1a,b ). Quantification of the centromere/cytoplasm ratio of Borealin staining indicated a value of 4.5±1.2 (average±s.d.) for Borealin 1–280 . In contrast, this ratio was significantly lower for both Borealin 1–221 (2.0±0.4, P <0.001 using a Student’s t -test) and Borealin 1–110 (1.7±0.3, P <0.001). Punctate staining of truncated forms of Borealin was also observed when expressed in cells in which the endogenous protein was knocked down using a untranslated region-targeted short hairpin RNA (shRNA) ( Supplementary Fig. 1 ). When either Borealin 1–221 or Borealin 1–110 were expressed in cells with endogenous Borealin intact, the level of INCENP on chromosomes was significantly reduced compared with cells transfected with full-length Borealin ( Fig. 1b,c ). 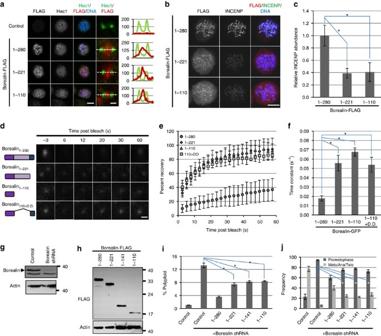Figure 1: Borealin structure–function analysis. (a) Immunofluorescence using antibodies to FLAG and Hec1 in HeLa M cells transfected with FLAG-tagged Borealin and then blocked in taxol. Whole-cell maximum projections (scale bar, 10 μm), individual sister kinetochores (scale bar, 0.5 μm) and line scans of Hec1 and Flag intensity in kinetochore images are shown. (b) Maximum projections from cells treated as inaand stained with antibodies against FLAG and INCENP (scale bar, 10 μm). (c) Intensity of INCENP in the DNA area of greater than 30 cells. Pixel intensities in INCENP images are relative to the average level of INCENP in untransfected samples from the same experiment. Bars represent s.d. (d) Representative still images of GFP foci from FRAP experiments in nocodazole-arrested HeLa M cells after transient transfection with GFP-tagged Borealin truncations (scale bar, 1 μm). (e) Post-bleach recovery of GFP-Borealin measured by FRAP. Averages and s.d. of more than eight centromeres per condition are shown. (f) Average time-constant values of FRAP curves frome(see Methods). (g) Borealin knockdown in HeLa M cells after transient transfection with pBabePURO, and either empty pSUPER (control) or pSUPER-Borealin shRNA. Cell lysates obtained after puromycin selection to remove untransfected cells were analysed by western blotting with antibodies against Borealin and Actin. (h) Expression of FLAG-tagged Borealin truncations. HeLa M cells were transfected with pSUPER-Borealin shRNA, pBABEpuro along with FLAG-tagged forms of Borealin. FLAG and actin were detected by western analysis. (i) Percentage of cells with greater than 4N DNA content (polyploid). HeLa M cells were transfected with pSUPER-Borealin shRNA, pBABEpuro and FLAG-tagged Borealin, exposed to puromycin and analysed by flow cytometry for DNA content 4 days post transfection. (j) Frequency of mitotic phases in Borealin knockdown cells expressing truncated forms of Borealin. HeLa M cells were transfected with pSUPER-Borealin shRNA, a plasmid encoding H2BGFP and Borealin truncations. Three days post transfection, mitotic phases of GFP-positive cells were determined. Scoring was carried out in a blinded manner (n≥100 for each condition). Bars fromiandjrepresent s.e. from three independent transfections. In sectionsc,f,iandjthe asterisk (*) indicatesP<0.05 using a Student’st-test. Figure 1: Borealin structure–function analysis. ( a ) Immunofluorescence using antibodies to FLAG and Hec1 in HeLa M cells transfected with FLAG-tagged Borealin and then blocked in taxol. Whole-cell maximum projections (scale bar, 10 μm), individual sister kinetochores (scale bar, 0.5 μm) and line scans of Hec1 and Flag intensity in kinetochore images are shown. ( b ) Maximum projections from cells treated as in a and stained with antibodies against FLAG and INCENP (scale bar, 10 μm). ( c ) Intensity of INCENP in the DNA area of greater than 30 cells. Pixel intensities in INCENP images are relative to the average level of INCENP in untransfected samples from the same experiment. Bars represent s.d. ( d ) Representative still images of GFP foci from FRAP experiments in nocodazole-arrested HeLa M cells after transient transfection with GFP-tagged Borealin truncations (scale bar, 1 μm). ( e ) Post-bleach recovery of GFP-Borealin measured by FRAP. Averages and s.d. of more than eight centromeres per condition are shown. ( f ) Average time-constant values of FRAP curves from e (see Methods). ( g ) Borealin knockdown in HeLa M cells after transient transfection with pBabePURO, and either empty pSUPER (control) or pSUPER-Borealin shRNA. Cell lysates obtained after puromycin selection to remove untransfected cells were analysed by western blotting with antibodies against Borealin and Actin. ( h ) Expression of FLAG-tagged Borealin truncations. HeLa M cells were transfected with pSUPER-Borealin shRNA, pBABEpuro along with FLAG-tagged forms of Borealin. FLAG and actin were detected by western analysis. ( i ) Percentage of cells with greater than 4N DNA content (polyploid). HeLa M cells were transfected with pSUPER-Borealin shRNA, pBABEpuro and FLAG-tagged Borealin, exposed to puromycin and analysed by flow cytometry for DNA content 4 days post transfection. ( j ) Frequency of mitotic phases in Borealin knockdown cells expressing truncated forms of Borealin. HeLa M cells were transfected with pSUPER-Borealin shRNA, a plasmid encoding H2BGFP and Borealin truncations. Three days post transfection, mitotic phases of GFP-positive cells were determined. Scoring was carried out in a blinded manner ( n ≥100 for each condition). Bars from i and j represent s.e. from three independent transfections. In sections c , f , i and j the asterisk (*) indicates P <0.05 using a Student’s t -test. Full size image To better understand the elevated cytoplasmic staining of Borealin truncations and the reduced INCENP levels, we measured centromere-binding dynamics of green fluorescent protein (GFP)-tagged Borealin in nocodazole-arrested mitotic cells, which also exhibit punctate localization of Borealin truncations (our unpublished data). Full-length Borealin-GFP recovered to ∼ 40% of pre-bleach levels within 60 s with a rate constant of ∼ 0.020 s −1 ( Fig. 1d–f ). Borealin 1–110 recovered to ∼ 90% of pre-bleach levels with a rate constant of ∼ 0.068 s −1 ( Fig. 1d–f ). Similarly, Borealin 1–221 recovered to ∼ 90% of pre-bleach levels with a rate constant of 0.056 s −1 ( Fig. 1d–f ). A Borealin mutant in which its dimerization domain was fused to amino acids 1–110 (Borealin 110+DD ) recovered to ∼ 90% of pre-bleach levels with a rate constant of 0.054 s −1 ( Fig. 1d–f ). These observations suggest that although the N-terminus of Borealin is sufficient for localization to centromeres, the C-terminus suppresses dynamic exchange to maintain stable CPC binding at this location. Furthermore, because Borealin 1–221 and Borealin 1–110 behave similarly, the N-terminus likely plays a dominant role in localization under these conditions. Because all Borealin truncations could be detected at centromeres, we tested whether these mutants retained CPC function during mitosis. Cells were transfected with Borealin shRNA along with shRNA-resistant Borealin C-terminal truncations and analysed by western blotting to confirm knockdown ( Fig. 1g,h ) and by flow cytometry to determine DNA content ( Fig. 1i ). Borealin shRNA alone increased the percentage of polyploid cells to ∼ 13% compared with 1% in control cells, indicating impaired CPC function ( Fig. 1i ). Expression of full-length Borealin reduced the incidence of polyploidy to ∼ 3.5%, while expression of any Borealin truncation partially rescued the incidence of polyploidy to ∼ 8% ( Fig. 1i ). Next, we measured the frequency of mitotic phases in cells expressing Borealin shRNA, Borealin truncations and H2BGFP as a screenable marker. Borealin shRNA alone increased the percentage of prometaphase cells to ∼ 95% compared with ∼ 20% in control cells, indicating impaired mitotic progression and defective CPC function ( Fig. 1j ). Co-expression of full-length Borealin with Borealin shRNA reduced the percentage of prometaphase cells to 60% ( Fig. 1j ). Co-expression of any Borealin C-terminal truncation with Borealin shRNA only partially rescued the incidence of prometaphase cells to ∼ 75% ( Fig. 1j ). In both flow cytometry and microscopic scoring, full-length Borealin did not completely rescue the shRNA-induced defects ( Fig. 1i,j ). Western blotting shows that in the entire transfected population, Borealin 1–280 -FLAG is ∼ 30% higher than endogenous Borealin ( Supplementary Fig. 2a ). The fact that it does not completely rescue may be due to cell-to-cell heterogeneity in expression. Importantly, in this background, the truncated proteins retain some wild-type Borealin function. This partial function maps mainly to the N terminus rather than the central region. Also, the extreme C-terminal region containing the dimerization domain is essential for full binding and function of the CPC at centromeres. Borealin dimerization regulates CPC abundance at centromeres Despite localizing to centromeres, Borealin 1–221 exchanges rapidly, which likely reduces steady-state levels of centromere INCENP ( Fig. 1a–f ). We hypothesized that the behaviour of this truncated Borealin protein was due to loss of the dimerization domain, previously mapped to amino acids 224–280 (ref. 26 ). Despite the existence of an nuclear magnetic resonance structure, the role of Borealin dimerization in CPC localization or function has not been resolved. In particular, mutations at residue T230 in the dimerization domain can reduce Aurora B activity at centromeres. However, reduced Aurora B activity is observed with mutations that either stabilize (T230V) or destabilize (T230A) the dimer in vitro [26] . More likely, these mutations alter Borealin function by disrupting phosphorylation [26] . Therefore, we created FKBP fusions using Borealin 1–221 or Borealin 1–110 where dimerization of FKBP fusion proteins can be induced using the small molecule AP20187 (ref. 28 ). Adding AP20187 to HeLa M cells expressing the Borealin–FKBP fusions did not alter the total levels of the fusion proteins ( Supplementary Fig. 2b ). Borealin–FKBP fusions proteins were expressed in taxol-arrested HeLa cells, which were then cultured in the presence or absence of the homo-dimerizing agent AP20187. Immunofluorescence was performed to assess localization of haemagglutinin (HA)-tagged Borealin–FKBP fusions, as well as Survivin, INCENP and Aurora B. Similar to FLAG-tagged Borealin truncations, expression of Borealin 1–221 –FKBP–HA or Borealin 1–110 –FKBP–HA reduced the levels of all CPC proteins in the absence of AP20187 ( Fig. 2a–c ). Under these conditions, undimerized Borealin 1–110 –FKBP–HA was more difficult to detect at centromeres compared with Borealin 1–221 –FKBP–HA ( Fig. 2a,b ). Inducing dimerization of Borealin by adding AP20187 increased the centromere localization of Survivin, INCENP and Aurora B ( Fig. 2a–c ). The intensity of Borealin 1–221 –FKBP–HA was also significantly increased by AP20187 ( Supplementary Fig. 3 ). Rescue of Borealin and Survivin levels were observed whether AP20187 was added before or after cells entered mitosis ( Supplementary Fig. 3 ). Therefore, CPC dimerization enhances its localization to the centromere. 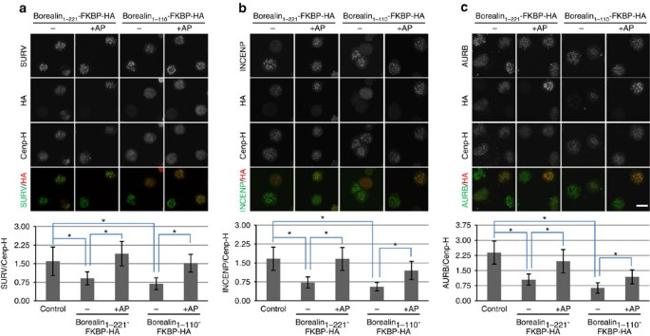Figure 2: Borealin dimerization regulates CPC abundance at centromeres. HeLa M cells were transfected with the indicated constructs and then exposed to thymidine for 24 h to synchronize in the S phase. At the time of thymidine removal, taxol was added in combination with AP20187 (+AP) or DMSO (—). Cells were fixed 16 h later and analysed by immunofluorescence. Intensity of centromere staining of Survivin (a), INCENP (b) and Aurora B (c) was quantified relative to the kinetochore marker CenpH (scale bar, 20 μm). Bars represent s.d. from averages of at least 50 centromere signals from 10 different cells per condition. *P<0.05 using a Student’st-test. Figure 2: Borealin dimerization regulates CPC abundance at centromeres. HeLa M cells were transfected with the indicated constructs and then exposed to thymidine for 24 h to synchronize in the S phase. At the time of thymidine removal, taxol was added in combination with AP20187 (+AP) or DMSO (—). Cells were fixed 16 h later and analysed by immunofluorescence. Intensity of centromere staining of Survivin ( a ), INCENP ( b ) and Aurora B ( c ) was quantified relative to the kinetochore marker CenpH (scale bar, 20 μm). Bars represent s.d. from averages of at least 50 centromere signals from 10 different cells per condition. * P <0.05 using a Student’s t -test. Full size image Haspin maintains the inner centromere CPC pool CPC localization to centromeres overlaps with two histone modifications, pH3 T3 and pH2A T120 , which in turn are regulated by Aurora B, Mps1, Bub1 and Haspin [17] , [18] , [19] . Disrupting Mps1 or Aurora B using inhibitors or RNA interference before mitotic entry reduces CPC localization to the centromere, indicating that these kinases are required to initially establish this localization [29] , [30] . Interestingly, centromere localization of Aurora B was not affected in cells exposed to reversine, a potent inhibitor of Mps1, when cells were previously arrested in mitosis with nocodazole [31] , [30] . To further investigate the role of pH2A T120 and pH3 T3 in maintaining CPC localization in mitotic cells, we used Aurora B, Mps1 or Haspin kinase inhibitors to correlate pH2A T120 and pH3 T3 levels with CPC localization. Inhibiting Aurora B with ZM447439 in nocodazole-arrested cells reduced pH2A T120 levels by ∼ 92% and pH3 T3 levels by ∼ 72% ( Fig. 3a,b ). Borealin and Aurora B were still detected at centromeres in ZM447439-treated cells ( Fig. 3c,d ), and analysis of image intensity in the region defined by DNA staining showed no significant reduction in either Borealin or Aurora B in response to this inhibitor ( Fig. 3e ). Inhibiting Mps1 after cells were arrested in mitosis with nocodazole also had no significant influence on whole-chromatin intensity of Borealin or Aurora B ( Fig. 3e ), despite a ∼ 92% reduction in pH2A T120 with no significant change in pH3 T3 levels ( Fig. 3a,b ). On the other hand, inhibiting Haspin with 5-iodotubercidin (5Itu) reduced the whole-chromatin intensity of Borealin and Aurora B by ∼ 60% coincident with a major reduction in pH3 T3 levels ( Fig. 3a,b,e ). We repeated these inhibitor treatments and quantified intensity of all core CPC members at individual centromeres in relation to the kinetochore marker CenpH. Aurora B, Borealin, INCENP and Survivin were unchanged in cells exposed to either reversine or ZM447439, whereas 5Itu significantly reduced all four proteins ( Supplementary Fig. 4a,b ). As a measure of CPC integrity, we measured co-immunoprecipitation of Survivin with Borealin. 5Itu treatment had no effect on this interaction, suggesting that the decrease in staining by immunofluorescence is not due to complete disassembly of the CPC ( Supplementary Fig. 2c ). We cannot rule out partial disassembly under these conditions. 5Itu can inhibit Haspin and other kinases including PKC, PKA, CK1 and CK2. The inhibitors chelerythrine chloride (PKC), H89 (PKA), D4476 (CK1) and TBB (CK2) had no effect on CPC localization during mitosis (our unpublished data). Furthermore, all CPC subunits were dispersed from centromeres in cells blocked in taxol and then exposed to the Haspin inhibitor CHR6494, which is structurally distinct from 5Itu, nevertheless showing similar effects as 5Itu ( Supplementary Fig. 5a ). These results suggest that Haspin is the relevant target of 5Itu with respect to CPC targeting to the centromere. In addition, Haspin inhibitors reduced CPC localization whether cells are blocked in nocodazole or taxol. Loss of Borealin at the centromere was also observed when either 5Itu or CHR6494 was added as cells were entering mitosis in the absence of spindle poisons, suggesting that this effect does not rely on spindle disruption ( Supplementary Fig. 5b ). 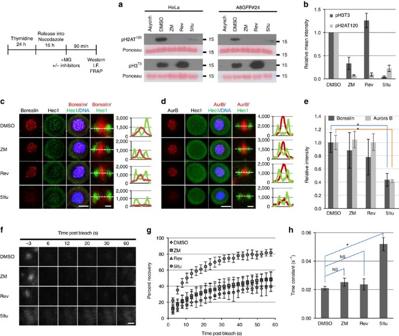Figure 3: Inner centromere localization of Borealin is regulated by Haspin kinase activity. HeLa M cells were synchronized and treated as shown in the schematic. Briefly, cells were released from a thymidine block in the presence of nocodazole to synchronously block them in mitosis. Mitotic cells were then exposed to MG132 to prevent mitotic exit and either DMSO, ZM447439 (ZM), reversine (Rev) or 5Itu. Ninety minutes after adding MG132 with or without inhibitors, cells were analysed by western blotting (a,b), immunofluorescence (IF) (c–e) or FRAP (f–h). (a) Western blot analysis of histone extracts. Histones were extracted and analysed by western blotting with the antibodies against pH2AT120and pH3T3. Ponceau S staining served as a loading control. Asynchronously growing cells (Asynch) were used as a negative control. (b) Quantification of band intensities from three independent western blots prepared as ina. (c,d) Maximum projections of HeLa M cells treated as described in the schematic. IF was performed using antibodies to either Borealin or Aurora B and Hec1. Hoechst was used to visualize DNA. Whole-cell maximum projections (scale bar, 10 μm) are shown with close-up images and line scans of individual sister kinetochores/centromeres from a single plane to the right (scale bar, 0.5 μm). (e) Quantification of the relative level of Borealin or Aurora B intensity in the DNA area of max projections fromcandd, respectively. Greater than 30 cells were quantified. (f) Representative still images of single centromeres from A8GFP#24 cells stably expressing Borealin-GFP treated as shown in the schematic (scale bar, 1 μm). (g) Post-recovery kinetics of Borealin-GFP under the indicated conditions. More than eight centromeres per condition were averaged in a single experiment. (h) The average time-constant values of FRAP curves fromg(see Methods). Inb,eandh, bars represent s.d. and the asterisk (*) indicatesP<0.05 using a Student’st-test. NS, not significant. Figure 3: Inner centromere localization of Borealin is regulated by Haspin kinase activity. HeLa M cells were synchronized and treated as shown in the schematic. Briefly, cells were released from a thymidine block in the presence of nocodazole to synchronously block them in mitosis. Mitotic cells were then exposed to MG132 to prevent mitotic exit and either DMSO, ZM447439 (ZM), reversine (Rev) or 5Itu. Ninety minutes after adding MG132 with or without inhibitors, cells were analysed by western blotting ( a , b ), immunofluorescence (IF) ( c – e ) or FRAP ( f – h ). ( a ) Western blot analysis of histone extracts. Histones were extracted and analysed by western blotting with the antibodies against pH2A T120 and pH3 T3 . Ponceau S staining served as a loading control. Asynchronously growing cells (Asynch) were used as a negative control. ( b ) Quantification of band intensities from three independent western blots prepared as in a . ( c , d ) Maximum projections of HeLa M cells treated as described in the schematic. IF was performed using antibodies to either Borealin or Aurora B and Hec1. Hoechst was used to visualize DNA. Whole-cell maximum projections (scale bar, 10 μm) are shown with close-up images and line scans of individual sister kinetochores/centromeres from a single plane to the right (scale bar, 0.5 μm). ( e ) Quantification of the relative level of Borealin or Aurora B intensity in the DNA area of max projections from c and d , respectively. Greater than 30 cells were quantified. ( f ) Representative still images of single centromeres from A8GFP#24 cells stably expressing Borealin-GFP treated as shown in the schematic (scale bar, 1 μm). ( g ) Post-recovery kinetics of Borealin-GFP under the indicated conditions. More than eight centromeres per condition were averaged in a single experiment. ( h ) The average time-constant values of FRAP curves from g (see Methods). In b , e and h , bars represent s.d. and the asterisk (*) indicates P <0.05 using a Student’s t -test. NS, not significant. Full size image To further investigate the role of pH2A T120 and pH3 T3 in CPC localization, fluorescence recovery after photobleaching (FRAP) was performed in nocodazole-arrested cells stably expressing full-length Borealin-GFP (A8GFP#24) in the presence or absence of Aurora B, Mps1 or Haspin inhibitors. As expected from previous studies, Borealin-GFP exchanged slowly at centromeres in control cells (exposed to dimethylsulphoxide (DMSO)), recovering to ∼ 40% of pre-bleach levels within a 60-s time window and a rate constant of 0.02 s −1 ( Fig. 3f–h ) [32] . Inhibiting Aurora B with ZM447439 (ZM) or Mps1 with reversine (Rev) did not significantly change the kinetics of Borealin-GFP recovery at centromeres ( Fig. 3f–h ). Inhibiting Haspin with 5Itu significantly increased the post-bleach recovery kinetics of Borealin-GFP, which recovered ∼ 85% of pre-bleach levels with a rate constant of 0.05 s −1 in a 60-s time window ( Fig. 3f–h ). These results suggest that stable association of Borealin with inner centromeres is regulated by Haspin kinase activity, but relatively unaffected by Aurora B or Mps1 inhibitors when cells have entered mitosis. Haspin inhibition reveals a kinetochore-proximal CPC pool Despite a major reduction in all CPC family members in response to 5Itu, residual staining is consistently observed. More detailed confocal imaging revealed that residual Borealin was observed in a kinetochore-proximal location ( Fig. 4a ). This pattern was observed in cells blocked either in nocodazole or taxol and whether 5Itu was added before or after cells had entered mitosis ( Fig. 4a,b ). Different kinetochore pairs in the same cell showed variation in the exact pattern of Borealin staining after 5Itu treatment; however, it was not uncommon to observe very close overlap with kinetochore markers ( Fig. 4b ; Supplementary Fig. 6 ). Careful analysis of nocodazole-arrested cells not exposed to 5Itu also revealed some kinetochore pairs with low levels of Borealin at or near kinetochores ( Fig. 4a ; column labelled ‘DMSO’). In general, this pool was difficult to discern due to high levels of inner centromere staining. Additional studies showed that Aurora B and Survivin could be detected in a kinetochore-proximal location in cells blocked in mitosis with taxol and then exposed to 5Itu ( Supplementary Fig. 7 ). Furthermore, all four core CPC family members showed a kinetochore-proximal staining pattern after 5Itu treatment that could be modulated by overexpression of truncated forms of Borealin (see below). 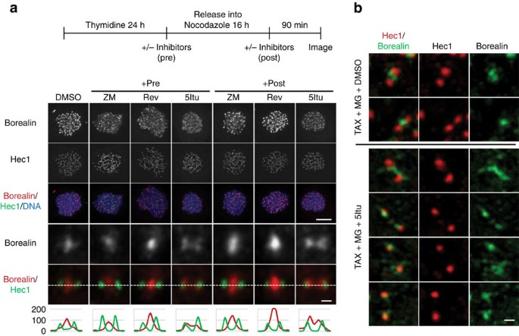Figure 4: Kinetochore-proximal Borealin pool observed after Haspin inhibition. (a) Borealin localization compared with Hec1. Cells were prepared as shown in the schematic. Maximum projection images of nocodazole-arrested HeLa M cells treated with the indicated inhibitors either before (+pre) or after (+post) mitotic entry are shown. Immunofluorescence was performed using antibodies against endogenous Borealin and Hec1. Examples of whole-cell maximum projections (scale bar, 10 μm) are shown. Close-up images and line scans of individual sister kinetochores/centromeres from a single plane are at the bottom (scale bar, 0.5 μm). (b) Co-localization of Borealin and Hec1 in taxol-arrested cells exposed to 5Itu. HeLa M cells were exposed to taxol for 6 h, and then with MG132 with or without 5Itu. Immunofluorescence was carried out 90 min post 5Itu addition. Confocal images were obtained with a 0.1-μm z-step followed by deconvolution using AutoQuant X3 software. Projection images are shown (scale bar, 0.5 μm). Figure 4: Kinetochore-proximal Borealin pool observed after Haspin inhibition. ( a ) Borealin localization compared with Hec1. Cells were prepared as shown in the schematic. Maximum projection images of nocodazole-arrested HeLa M cells treated with the indicated inhibitors either before (+pre) or after (+post) mitotic entry are shown. Immunofluorescence was performed using antibodies against endogenous Borealin and Hec1. Examples of whole-cell maximum projections (scale bar, 10 μm) are shown. Close-up images and line scans of individual sister kinetochores/centromeres from a single plane are at the bottom (scale bar, 0.5 μm). ( b ) Co-localization of Borealin and Hec1 in taxol-arrested cells exposed to 5Itu. HeLa M cells were exposed to taxol for 6 h, and then with MG132 with or without 5Itu. Immunofluorescence was carried out 90 min post 5Itu addition. Confocal images were obtained with a 0.1-μm z-step followed by deconvolution using AutoQuant X3 software. Projection images are shown (scale bar, 0.5 μm). Full size image The kinetochore-proximal pool of Borealin revealed after Haspin inhibition is similar to the localization pattern of residual pH2A T120 ( Fig. 5a ) [18] , [33] . Thus, immunofluorescence was performed in nocodazole-arrested A8GFP#24 cells to assess both pH2A T120 and Borealin-GFP localization in the same cells after inhibiting Aurora B, Mps1 and Haspin. A8GFP#24 cells were used due to the availability of monoclonal antibodies to GFP, but not Borealin. As expected, Borealin-GFP localized between sister kinetochores despite a major reduction in pH2A T120 when Aurora B or Mps1 were inhibited ( Fig. 5b ). Borealin-GFP at inner centromeres was reduced after inhibiting Haspin and the residual pool of Borealin formed two peaks, which partially co-localized with pH2A T120 ( Fig. 5b ). 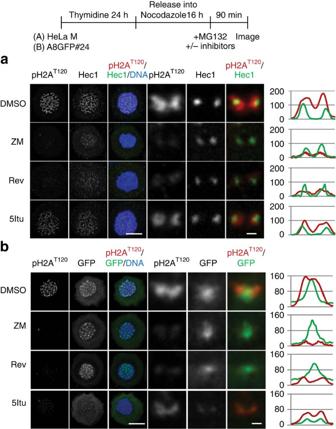Figure 5: Kinetochore localization of Borealin overlaps with pH2AT120. HeLa M cells or a stable clone of HeLa M expressing Borealin-GFP (A8GFP#24) were treated as indicated in the schematic. Briefly, cells were released from a thymidine block in the presence of nocodazole. Sixteen hours later when most cells were blocked in mitosis, DMSO, ZM447439 (ZM), reversine (Rev) or 5Itu was added. MG132 was added under all conditions to block mitotic exit. Cells were fixed 90 min after inhibitors were added, stained with the indicated antibodies and analysed by confocal microscopy. (a) Partial overlap between pH2AT120with Hec1 in HeLa M cells exposed to 5Itu. Examples of maximum projections are shown (scale bar, 10 μm). Close-up images and line scans of individual sister kinetochores/centromeres from a single plane are to the right (scale bar, 0.5 μm). (b) Partial co-localization of Borealin-GFP with pH2AT120in cells blocked in 5Itu. A8GFP#24 cells were treated as indicated in the schematic and stained with antibodies to GFP to enhance detection as well as pH2AT120. Examples of maximum projections (scale bar, 10 μm) and kinetochore pairs (scale bar, 0.5 μm) are shown. Figure 5: Kinetochore localization of Borealin overlaps with pH2A T120 . HeLa M cells or a stable clone of HeLa M expressing Borealin-GFP (A8GFP#24) were treated as indicated in the schematic. Briefly, cells were released from a thymidine block in the presence of nocodazole. Sixteen hours later when most cells were blocked in mitosis, DMSO, ZM447439 (ZM), reversine (Rev) or 5Itu was added. MG132 was added under all conditions to block mitotic exit. Cells were fixed 90 min after inhibitors were added, stained with the indicated antibodies and analysed by confocal microscopy. ( a ) Partial overlap between pH2A T120 with Hec1 in HeLa M cells exposed to 5Itu. Examples of maximum projections are shown (scale bar, 10 μm). Close-up images and line scans of individual sister kinetochores/centromeres from a single plane are to the right (scale bar, 0.5 μm). ( b ) Partial co-localization of Borealin-GFP with pH2A T120 in cells blocked in 5Itu. A8GFP#24 cells were treated as indicated in the schematic and stained with antibodies to GFP to enhance detection as well as pH2A T120 . Examples of maximum projections (scale bar, 10 μm) and kinetochore pairs (scale bar, 0.5 μm) are shown. Full size image Borealin dimerization is needed for kinetochore localization To further investigate the kinetochore-proximal pool of Borealin, we tested the effect of inducible dimerization on this localization pattern. Immunofluorescence was performed using antibodies to HA to detect Borealin–FKBP fusions along with the kinetochore protein Hec1. Taxol-arrested HeLa M cells expressing Borealin 1–221 –FKBP–HA or Borealin 1–110 –FKBP–HA were incubated in the presence or absence of the dimerizing agent AP20187 after inhibiting Haspin. In observations of at least 50 transfected cells, we failed to detect punctate staining of either Borealin 1–221 –FKBP–HA or Borealin 1–110 –FKBP–HA in Haspin-inhibited cells in the absence of the dimerizer AP20187 (for examples, see Fig. 6 ). In the presence of AP20187, Borealin 1–221 –FKBP–HA, but not Borealin 1–110 –FKBP–HA, was detectable as punctate foci that co-localized with Hec1 ( Fig. 6 ). Therefore, the central region of Borealin and dimerization are essential for CPC localization to the kinetochore when Haspin is inhibited. Next, we quantified the intensities of CPC proteins relative to CenpH in 5Itu-treated cells transfected with Borealin 1–221 –FKBP–HA. INCENP, Survivin and Aurora B were detected near kinetochores in untransfected, 5Itu-treated cells ( Fig. 7 ). Overexpressing Borealin 1–221 –FKBP–HA in the absence of AP20187 reduced the kinetochore-proximal staining of all three CPC proteins, a defect that was rescued by addition of AP20187 ( Fig. 7 ). 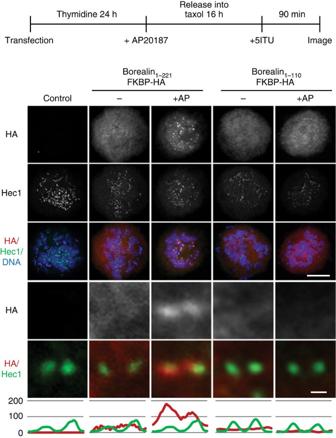Figure 6: Borealin dimerization is essential for localization near the kinetochore. HeLa M cells were transiently transfected with Borealin–FKBP fusions, synchronized as shown and exposed to the homo-dimerizing agent AP20187 (+AP) or DMSO (—). All samples include 5Itu to reveal the kinetochore pool. Immunofluorescence was carried out using antibodies to HA to detect the Borealin–FKBP fusions, as well as Hec1 to stain the kinetochore. Examples of maximum projection images are shown in the top three rows (scale bar, 10 μm). Close-up images and line scans of individual sister kinetochores/centromeres from a single plane are also shown (scale bar, 0.5 μm). Figure 6: Borealin dimerization is essential for localization near the kinetochore. HeLa M cells were transiently transfected with Borealin–FKBP fusions, synchronized as shown and exposed to the homo-dimerizing agent AP20187 (+AP) or DMSO (—). All samples include 5Itu to reveal the kinetochore pool. Immunofluorescence was carried out using antibodies to HA to detect the Borealin–FKBP fusions, as well as Hec1 to stain the kinetochore. Examples of maximum projection images are shown in the top three rows (scale bar, 10 μm). Close-up images and line scans of individual sister kinetochores/centromeres from a single plane are also shown (scale bar, 0.5 μm). 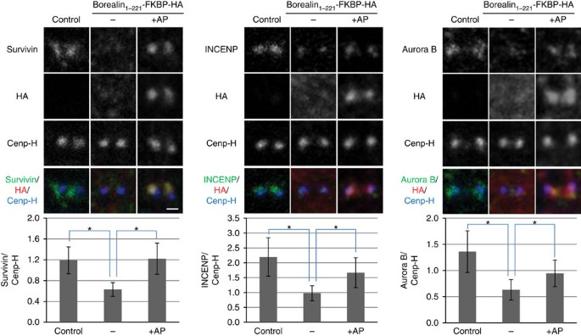Figure 7: Monomeric but not dimeric Borealin1–221–FKBP reduces CPC subunits at the kinetochore. HeLa M cells were synchronized and treated as shown in the schematic toFig. 5. However, when fixed, the cells were stained with antibodies to Survivin, INCENP, Aurora B, CenpH to mark the kinetochore and HA to detect the Borealin–FKBP fusions. All cells were exposed to 5Itu (added as indicated inFig. 5) to remove the inner centromere pool and reveal the kinetochore pool. Examples of close-up confocal images of individual sister kinetochores/centromeres are shown for all conditions (scale bar, 0.5 μm). Intensity of CPC family members was quantified and is shown relative to CenpH at individual kinetochores. At least 50 kinetochores from 10 different cells were analysed. Bars represent s.d. *P<0.05 using a Student’st-test. Full size image Figure 7: Monomeric but not dimeric Borealin 1–221 –FKBP reduces CPC subunits at the kinetochore. HeLa M cells were synchronized and treated as shown in the schematic to Fig. 5 . However, when fixed, the cells were stained with antibodies to Survivin, INCENP, Aurora B, CenpH to mark the kinetochore and HA to detect the Borealin–FKBP fusions. All cells were exposed to 5Itu (added as indicated in Fig. 5 ) to remove the inner centromere pool and reveal the kinetochore pool. Examples of close-up confocal images of individual sister kinetochores/centromeres are shown for all conditions (scale bar, 0.5 μm). Intensity of CPC family members was quantified and is shown relative to CenpH at individual kinetochores. At least 50 kinetochores from 10 different cells were analysed. Bars represent s.d. * P <0.05 using a Student’s t -test. Full size image Experiments with Borealin-GFP suggest that Borealin co-localizes with pH2A T120 in 5Itu-treated cells ( Fig. 5a ). We repeated this co-localization experiment using the inducible FKBP-dimerization system. As before, undimerized Borealin 1–221 –FKBP was dispersed in the cytoplasm after 5Itu treatment ( Fig. 8 ). Interestingly, this truncated protein also dispersed the residual pH2A T120 in 5Itu-treated cells ( Fig. 8 ). Adding AP20187 rescued both punctate Borealin 1–221 –FKBP and pH2A T120 staining ( Fig. 8 ). We also tested the effect of combined treatment with 5Itu and either reversine or ZM447439 on localization of the dimerized Borealin 1–221 –FKBP. Similarly to our results with FLAG-tagged proteins, adding either reversine or ZM447439 appeared to uncouple Borealin localization from pH2A T120 , in that Borealin was still partially punctate, while the histone modification was dispersed ( Fig. 8 ). 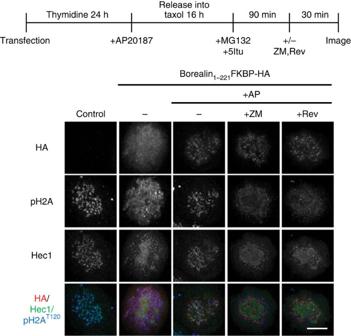Figure 8: Kinetochore Borealin can be uncoupled from pH2AT120. HeLa M cells were synchronized and treated as shown in the schematic. Briefly, cells were transfected with the indicated Borealin–FKBP and synchronously released into a taxol block. All cells received AP20187 to induce dimerization. Once cells were in mitosis, 5Itu was added for 90 min. Then, either ZM447439 (ZM) or reversine (Rev) was added for an additional 30 min before cells were fixed. Immunofluorescence was carried out with antibodies to pH2AT120, Hec1 or HA to detect the Borealin–FKBP fusion. Maximum projection images are shown (scale bar, 10 μm). Figure 8: Kinetochore Borealin can be uncoupled from pH2A T120 . HeLa M cells were synchronized and treated as shown in the schematic. Briefly, cells were transfected with the indicated Borealin–FKBP and synchronously released into a taxol block. All cells received AP20187 to induce dimerization. Once cells were in mitosis, 5Itu was added for 90 min. Then, either ZM447439 (ZM) or reversine (Rev) was added for an additional 30 min before cells were fixed. Immunofluorescence was carried out with antibodies to pH2A T120 , Hec1 or HA to detect the Borealin–FKBP fusion. Maximum projection images are shown (scale bar, 10 μm). Full size image Checkpoint function of a kinetochore-proximal CPC pool The role of CPC in error correction is thought to rely on its inner centromere localization, providing a spatially restricted gradient of Aurora B phosphorylation [15] . On the other hand, studies in budding yeast suggest that the CPC may contribute to error correction even when displaced from the inner centromere [16] . Also, mitotic arrest induced by taxol is much more efficiently abrogated by Aurora B inhibitors compared with the Haspin inhibitor 5Itu [34] . We hypothesized that residual CPC recruited to the kinetochore-proximal pool in Haspin-inhibited cells contributes to continuous error correction in taxol leading to persistent mitotic arrest. Our experiments so far suggest that monomeric CPC can only interact with the centromere if Haspin is active. For example, Borealin 1–221 -FLAG still localizes to centromeres in untreated cells ( Fig. 1a ), whereas monomeric Borealin 1–221 –FKBP fails to localize in 5Itu-treated cells ( Figs 6 , 7 , 8 ). In addition, monomeric Borealin 1–221 –FKBP displaces CPC from the kinetochore-proximal pool ( Fig. 7 ). Therefore, we used monomeric Borealin 1–221 -GFP to displace CPC from the kinetochore-proximal pool in cells simultaneously exposed to 5Itu (to remove the inner centromere pool). In this manner we could test whether the kinetochore-proximal pool contributes to the taxol arrest. Cells expressing full-length Borealin-GFP or Borealin 1–221 -GFP were synchronized into taxol, and the mitotic index and fraction of cells that escaped mitosis were monitored by time-lapse microscopy following exposure to 5Itu. In cells expressing full-length Borealin-GFP, 5Itu reduced the mitotic index to ∼ 35% compared with ∼ 49% in DMSO-treated controls ( Fig. 9 ). Also, ∼ 25% of cells escaped mitosis after 5Itu treatment compared with ∼ 7% escape in DMSO-treated cells. Inhibiting Haspin in cells expressing Borealin 1–221 -GFP decreased the mitotic index to ∼ 20% compared with ∼ 41% in DMSO-treated cells. Moreover, ∼ 40% of Borealin 1–221 -GFP expressing cells escaped mitosis in 5Itu compared with ∼ 12% escape in DMSO controls ( Fig. 7b ). Importantly, in the presence of 5Itu, overexpressing Borealin 1–221 -GFP weakened the mitotic arrest compared with cells overexpressing full-length Borealin. These results suggest that the kinetochore-proximal CPC pool plays an important role in maintaining the mitotic arrest induced by taxol. 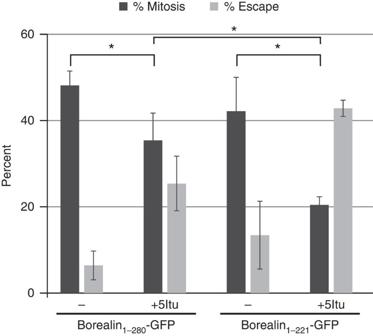Figure 9: Checkpoint function of a kinetochore-proximal CPC pool. HeLa M cells were transfected and synchronized into the S phase by 24-h treatment with 2 mM thymidine. Following synchronization, cells were released into taxol for 16 h and time-lapse imaging was performed immediately after adding either DMSO (—) or 5Itu. The percentage of Borealin-GFP-expressing cells remaining in mitosis or having escaped mitosis by 15-h after 5Itu treatment is shown. Bars represent s.e. from three independent transfections. *P<0.05 from a Student’st-test. Figure 9: Checkpoint function of a kinetochore-proximal CPC pool. HeLa M cells were transfected and synchronized into the S phase by 24-h treatment with 2 mM thymidine. Following synchronization, cells were released into taxol for 16 h and time-lapse imaging was performed immediately after adding either DMSO (—) or 5Itu. The percentage of Borealin-GFP-expressing cells remaining in mitosis or having escaped mitosis by 15-h after 5Itu treatment is shown. Bars represent s.e. from three independent transfections. * P <0.05 from a Student’s t -test. Full size image Correcting improper kinetochore–microtubule interactions during mitosis is essential to prevent aneuploidy, a common characteristic of cancer cells. Centromere-localized CPC is critical for an error correction mechanism that activates the SAC to prevent aneuploidy [15] , [35] . Our results have uncovered important details of CPC localization and function at the centromere. Borealin 1–110 and Borealin 1–221 localize to centromeres but exchange more rapidly than the full-length protein. Both proteins retain the N-terminal alpha helices needed to interact with INCENP and Survivin. These results suggest that Borealin 1–110 and Borealin 1–221 assemble a monomeric CPC that interacts with the centromere via a single binding site for pH3 T3 provided by Survivin ( Fig. 10 ). Borealin 1–221 contains all the Cdk1 phosphorylation sites required to bind to Sgo1/2. In principle, a CPC monomer created with Borealin 1–221 might simultaneously bind pH3 T3 via Survivin and pH2A T120 via Sgo1/2. Our data argue that if this is the case, the contribution of pH2A T120 to the binding energy must be minimal. Otherwise, Borealin 1–221 would show significantly slower exchange than Borealin 1–110 . 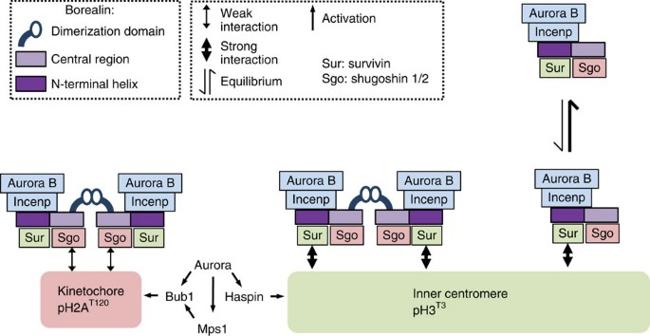Figure 10: Model for the role of dimerization in CPC interactions with the centromere. Dimeric CPC stably binds at inner centromeres possibly via two Survivin–pH3T3interactions mediated by Borealin dimerization. Removing the dimerization domain of Borealin results in rapid exchange at inner centromeres since monomeric CPC might only contact a single pH3T3molecule. When endogenous Borealin is knocked down, Borealin mutants lacking dimerization transiently associate with the centromere to provide partial function. However, when endogenous Borealin is present, dimerization-defective mutants compete for other CPC family members to increase their exchange and act as dominant negatives. At the kinetochore, dimeric CPC binds with a high rate of turnover potentially via dual pH2AT120–Sgo1/2 interactions. These kinetochore interactions are too weak to allow association in the context of a monomeric CPC. According to the prevailing model of CPC targeting, CPC interacts simultaneously with pH3T3via Survivin and pH2AT120via Sgo1/2. Our results do not preclude simultaneous binding, but do suggest that pH3T3would contribute most of the binding energy if this binding mode occurs. Theoretically, CPC monomers or dimers could simultaneously interact with single pH3T3and pH2AT120. Figure 10: Model for the role of dimerization in CPC interactions with the centromere. Dimeric CPC stably binds at inner centromeres possibly via two Survivin–pH3 T3 interactions mediated by Borealin dimerization. Removing the dimerization domain of Borealin results in rapid exchange at inner centromeres since monomeric CPC might only contact a single pH3 T3 molecule. When endogenous Borealin is knocked down, Borealin mutants lacking dimerization transiently associate with the centromere to provide partial function. However, when endogenous Borealin is present, dimerization-defective mutants compete for other CPC family members to increase their exchange and act as dominant negatives. At the kinetochore, dimeric CPC binds with a high rate of turnover potentially via dual pH2A T120 –Sgo1/2 interactions. These kinetochore interactions are too weak to allow association in the context of a monomeric CPC. According to the prevailing model of CPC targeting, CPC interacts simultaneously with pH3 T3 via Survivin and pH2A T120 via Sgo1/2. Our results do not preclude simultaneous binding, but do suggest that pH3 T3 would contribute most of the binding energy if this binding mode occurs. Theoretically, CPC monomers or dimers could simultaneously interact with single pH3 T3 and pH2A T120 . Full size image Borealin 1–110 and Borealin 1–221 could partially replace endogenous Borealin in supporting progression through mitosis. This partial rescue suggests that slow exchange of the CPC at the centromere is required to properly coordinate chromosome attachment to the spindle. Rapid exchange is also consistent with the ability of truncated Borealin proteins to partially displace INCENP from the centromere. We hypothesized that these effects are the consequence of forming a monomeric CPC that presents half the number of binding sites for centromeric receptors, which spends more time in the cytoplasm with a resulting partial loss of function ( Fig. 10 ). To investigate this idea, the dimerization domain of Borealin was replaced with FKBP allowing inducible dimerization [28] , [36] , [37] . Borealin 1–221 –FKBP was localized to centromeres and the cytoplasm in the absence of the AP20187 dimerizer. These conditions also dispersed the CPC from the centromere. Addition of AP20187 rescued centromere localization of both Borealin 1–221 –FKBP and CPC, showing that dimerization is required for efficient association with the centromere ( Fig. 10 ). The Borealin 1–110 –FKBP fusion was difficult to detect at centromeres in the absence of AP20187, but still able to displace the CPC suggesting that the N-terminal triple-helical bundle is intact. AP20187 rescued Borealin 1–110 –FKBP, Aurora B, INCENP and Survivin providing more evidence that the central region of Borealin plays a minor role in inner centromere CPC targeting. In contrast, Borealin 110+DD displayed similar kinetics compared with fragments containing amino acids 1–110 or 1–221. We hypothesize that the two CPC arms must be a minimum distance to support dual interaction with the centromere. We used several approaches to correlate CPC localization and the known centromere receptors, pH3 T3 and pH2A T120 . For example, Mps1 inhibition reduced pH2A T120 by ∼ 92%, but did not affect pH3 T3 nor CPC localization or dynamics. CPC localization and Borealin dynamics were also unchanged in mitotic cells exposed to ZM447439, which reduced pH2A T120 by ∼ 92% and pH3 T3 by ∼ 72%. Therefore, CPC localization can be uncoupled from the majority of pH2A T120 and pH3 T3 if the inhibitors are added after cells enter mitosis. 5Itu was more efficient than either ZM447439 or reversine at reducing pH3 T3 and subsequently reduced all CPC family members at centromeres and increased Borealin centromere dynamics. Detailed confocal analysis of 5Itu-treated cells revealed a subpopulation of Borealin proximal to kinetochores. Analysis of Borealin–FKBP fusions showed that localization near the kinetochore only occurs when the CPC is dimerized and only when the central domain of Borealin implicated in pH2A T120 recognition is intact. We interpret this observation to indicate that a CPC dimer, but not monomer associates with two copies of a kinetochore-proximal target, which may be pH2A T120 . Presumably the monomeric CPC–kinetochore interaction is too weak to allow stable association via a single binding surface ( Fig. 10 ). Our FRAP experiments using full-length Borealin-GFP in 5Itu-treated cells showed a faster exchange than untreated cells. Most likely, this condition measures the exchange of the kinetochore-proximal CPC pool. The detection of CPC near the kinetochore may have important consequences for error correction. Chromosomes under tension show undetectable levels of CPC at the kinetochore (for examples, see refs 35 , 38 , 39 ). Our experiments have been carried out in the presence of spindle toxins, which may be responsible for the localization pattern observed. The presence of CPC members near kinetochores is not unprecedented, as phosphorylated Aurora B has been detected near kinetochores [40] , [41] . In any case, the kinetochore-proximal pool is most evident in cells exposed to 5Itu, which presumably removes most of the inner centromere pool bound to pH3 T3 . Considering the spatial gradient model of CPC function, even small amounts of kinetochore-localized CPC might have marked effects on microtubule binding and checkpoint activation. To test this idea we took advantage of monomeric Borealin 1–221 , which does not efficiently bind kinetochores when pH3 T3 is depleted by 5Itu. When Borealin 1–221 overexpression was combined with 5Itu, the taxol arrest was weaker than with either condition alone. 5Itu is likely inefficient due to residual CPC at the kinetochore. Borealin 1–221 in the absence of 5Itu still localizes to centromeres, likely via stronger binding of the monomer to pH3 T3 . This explains why this truncated protein is not an efficient dominant-negative as long as pH3 T3 is present. Combining Borealin 1–221 and 5Itu removes both the centromere and kinetochore pools of CPC to provide more efficient checkpoint override. Our inhibitor and staining studies combined with published literature are consistent with CPC binding to pH3 T3 at the inner centromere and possibly Sgo/pH2A T120 at the kinetochore [18] , [19] , [42] , [43] , [44] , [45] , [46] , [47] . However, several lines of evidence argue against Sgo/pH2A T120 as the receptor for residual CPC found at the kinetochore. For example, Borealin localization can be uncoupled from pH2A T120 when cells are exposed to 5Itu in combination with either reversine or ZM447439 ( Fig. 8 ). Also, a recent study has uncovered a Borealin–HP1 interaction that may contribute to kinetochore localization [48] . Furthermore, under conditions of low inter-kinetochore tension, such as during a nocodazole block, Sgo1 binds to cohesin in place of pH2A T120 (ref. 33 ) In the context of our results, Sgo1/2 binding to cohesin is unlikely to explain the kinetochore-proximal localization of Borealin in 5Itu-treated cells simply due to its location near the kinetochore and not inner centromere. In addition, in untreated cells the inner centromere localization of Borealin truncations we have observed occur with the minimal INCENP/Survivin-binding region, and most likely occur via binding to pH3 T3 . It is also possible that CPC is recruited to pH2A T120 at the kinetochore in an Sgo1/2-independent manner. In conclusion, Borealin dimerization is critical for suppressing dynamic exchange at inner centromeres, localization to kinetochores and maximum function of the CPC. In addition, monomeric CPC can be targeted to the inner centromere presumably via pH3 T3 . Although CPC binds to a kinetochore-proximal location, this only occurs if CPC is dimerized. The role of dimerization appears to be to simply double the interaction surfaces of CPC with centromere receptors to provide tighter binding and full function. Cell culture and drug treatments Cells were grown in Dulbecco’s minimal essential medium (Gibco) with penicillin/streptomycin and 10% fetal bovine serum in a humidified atmosphere of 10% CO 2 at 37 °C. All experiments were performed with HeLa M cells, a sub-line of HeLa originally obtained from Dr G.C. Sen [49] . FRAP experiments in Fig. 3 were performed using a HeLa M clone stably transfected with Borealin-GFP (our unpublished data). Transient transfections were performed using either XtremeGene (Roche) or Expressfect (Denville Scientific Inc.) with similar results. Synchronization of cells was performed by treating cells with 2 mM thymidine (Sigma Aldrich) for 24 h followed by release into either 3.3 μM nocodazole (Sigma Aldrich) or 0.5 μM taxol (Cayman Chemical) to arrest cells in mitosis. The proteasome inhibitor MG132 (Cayman chemical) was used at a concentration of 20 μM and kinase inhibitors were used at previously determined effective concentrations: 2.5 μM ZM447439 (AstraZeneca), 2 μM reversine (Calbiochem), 2 μM 5Itu (Santa Cruz) and 1 μM CHR6494 (EMD Millipore). Finally, cell selection was accomplished using puromycin at 1 μg μl −1 (Invitrogen). In Borealin–FKBP experiments the small molecule AP20187 was used at 500 nM (Clonetech). Construction of Borealin truncations and fusions Borealin truncation mutants were constructed by amplifying the corresponding regions of a complementary DNA (cDNA) encoding human Borealin by PCR. The PCR products encoding a FLAG-tag at the C terminus were TOPO cloned into pcDNA 3.2 (Invitrogen) [20] , [50] . A Borealin fusion was constructed by amplifying regions of Borealin cDNA corresponding to amino acids 1–110 and 221–280 with SpeI restriction sites at the 3′ and 5′ ends. The PCR products were digested with SpeI followed by gel purification and ligation. The ligated product was Gateway cloned into pDEST47 (Invitrogen). Borealin–FKBP fusions were constructed by amplifying regions of Borealin cDNA corresponding to amino acids 2–110 or 2–221 with XbaI and SpeI restriction sites at the 3′ and 5′ ends, respectively. The PCR products were digested with SpeI and XbaI followed by gel purification and ligation into XbaI-digested pC 4 -F v 1E (ARIAD Pharmaceuticals). All constructs were confirmed by sequencing. Primer sequences are available upon request. Immunofluorescence microscopy For immunofluorescence microscopy, HeLa M cells were grown on coverslips followed by transient transfection where indicated. Following synchronization and drug treatment, cells were fixed with 2% formaldehyde/PBS for 10 min then permeabilized with 150 mM NaCl, 10 mM Tris (pH 7.7), 0.1% Triton-X-100 (v/v) and 0.1% BSA (w/v) for 9 min [51] . Fixed cells were blocked with PBS containing 0.1% BSA for 16 h at 4 °C followed by detection with the following antibodies where indicated: rabbit anti-FLAG (M2; Sigma), mouse anti-Hec1 (9G3; Abcam), rabbit anti-Aurora B (H75; Santa Cruz), mouse anti-INCENP (58-217; Millipore), mouse anti-Survivin (6E4; Cell signaling), rabbit anti-HA (C29F4; Cell signaling), rabbit anti-pH3 T3 (9714S; Cell Signaling) mouse anti-GFP (3E6; Invitrogen), rabbit pH2A T120 (61195; Active Motif) or affinity-purified rabbit anti-Borealin [52] . Some experiments included a rat anti-CenpH antibody to detect kinetochores (gift from Dr S.T. Liu) [53] . Conjugated secondary antibodies included goat-anti-mouse Alexafluor-488, goat-anti-rabbit Alexafluor-568 and goat anti-rat Alexafluor-647 (Invitrogen). Primary antibodies were generally diluted at either 1:100, 1:200 or 1:500 in PBS containing 0.1% BSA. The optimum dilution to reduce background and maintain the specific signal was determined separately for each antibody and usually repeated for each new lot. Within an experiment, antibody dilutions were always identical between samples. Secondary antibodies were diluted 1:500 in PBS plus 0.1% BSA. Coverslips were mounted using Vectashield (Vector Laboratories) and analysed using a Leica SP8 confocal microscope. Histone extraction and western blotting For western blot analysis of histone modifications, cell pellets were obtained after synchronization and drug treatment and histones were extracted as described [54] . Cell pellets were lysed in Nuclear Prep buffer containing 10 mM Tris pH 7.6, 150 mM NaCl, 1.5 mM MgCl 2 and 0.65% NP40 for 30 min on ice and then spun at 1,500 g for 10 min at 4 °C. Pelleted nuclei were then resuspended in RSB buffer containing 10 mM NaCl, 10 mM Tris-HCl pH 7.5, 3 mM MgCl 2 and 0.4 N sulfuric acid and incubated on ice for 30 min and then spun at maximum speed for 20 min at 4 °C. Trichloroacetic acid was added to the supernatant at 18% and incubated on ice for 30 min and then spun at maximum speed for 30 min at 4 °C. Pelleted histones were washed with acetone:HCl (99.5:0.5% v/v) then with 100% acetone followed by air drying. Histones were resuspended in H 2 O and separated by SDS–polyacrylamide gel electrophoresis and transferred to polyvinylidene difluoride membrane. The membrane was stained with Ponceau S to indicate loading and then probed with the following antibodies for western analysis: rabbit anti-pH3 T3 (Cell Signaling), rabbit anti-pH2A T120 (Abcam). Uncropped images of all western blots are shown in Supplementary Figs 8, 9 and 10 . Flow cytometry and analysis of mitotic progression For analysis of DNA content by flow cytometry, cells were transfected with pBabePURO, pSUPER-Borealin shRNA or pSUPER empty (control), and plasmids encoding FLAG-tagged Borealin truncations. Following 3 days of selection in 1 μg μl −1 puromycin, cells were collected by centrifugation at 2,000 g for 7 min at 4 °C and resuspended in PBS [55] . Cells were fixed in 70% ethanol at −20 °C for 16 h. Fixed cells were collected by centrifugation, resuspended in PBS and stained with 0.5 mg ml −1 of propidium iodide along with 5 μg ml −1 of RNAse A for 30 min. Cells were then analysed by flow cytometry using CellQuest and WinMDI software. Ten thousand cells were analysed for each sample. For Fig. 1g,h , cells were treated as above, however, cells were harvested and lysed in RIPA buffer and then lysates were separated by SDS–polyacrylamide gel electrophoresis and transferred to polyvinylidene difluoride for western blotting using rabbit anti-Borealin [52] , mouse anti-actin (Abcam) or rabbit anti-FLAG (Sigma). For experiments analysing mitotic progression in Fig. 1j , cells were transfected as above; however, pBabePURO was replaced with H2BGFP. Three days post transfection, live cells were imaged by fluorescence microscopy and mitotic stages quantified in a blinded manner (plates were coded by the person doing the transfection and a different person scored the mitotic stages). Fluorescence recovery after photobleaching (FRAP) For FRAP studies, cells were plated on glass-bottom 35-mm dishes (World Precision Instruments) followed by transfection and synchronization into mitosis. During imaging, cells were maintained at 37 °C at 5% CO 2 in a Tokai Hit Stage Top Incubator. Photobleaching and four-dimensional confocal microscopy were performed on a Leica SP8 system using the × 100 oil objective. GFP was excited with a 488-nm Argon laser (power varying from 0.05 to 0.1% at 70% maximum power). Individual centromeres were imaged by successive acquisition of 2.5-μm volumes at 0.5 μm per step along the z axis at a zoom factor of 10. Centromeres were bleached by five iterations of a full power laser and recovery was monitored every 2.616 s for ∼ 2 min post bleaching. Fluorescence intensities of bleached centromeres were acquired from the Leica AF software. After background subtraction, the mean intensity of the region prior to photobleaching was set at 100% and relative intensities at each time point were averaged for greater than eight centromeres from individual cells (averaged data set). Fit curves were generated by minimizing the χ 2 -value of the averaged data set, and a fit curve by adjusting parameters C, A and k (time constant) in the following equation using the Microsoft Excel Solver function: Average time constants were obtained by fitting individual FRAP curves and then averaging the time constants for each condition. Statistical analysis for all experiments in this paper involved pairwise comparisons using a two-tailed Student’s t -test. P values below 0.05 were considered to indicate significant differences. How to cite this article: Bekier, M. E. et al. Borealin dimerization mediates optimal CPC checkpoint function by enhancing localization to centromeres and kinetochores. Nat. Commun. 6:6775 doi: 10.1038/ncomms7775 (2015).